Silicon-in-silica spheres via axial thermal gradient in-fibre capillary instabilities The ability to produce small scale, crystalline silicon spheres is of significant technological and scientific importance, yet scalable methods for doing so have remained elusive. Here we demonstrate a silicon nanosphere fabrication process based on an optical fibre drawing technique. A silica-cladded silicon-core fibre with diameters down to 340 nm is continuously fed into a flame defining an axial thermal gradient and the continuous formation of spheres whose size is controlled by the feed speed is demonstrated. In particular, spheres of diameter <500 nm smaller than those produced under isothermal heating conditions are shown and analysed. A fibre with dual cores, p -type and n -type silicon, is drawn and processed into spheres. Spatially coherent break-up leads to the joining of the spheres into a bispherical silicon ‘ p – n molecule’. The resulting device is measured to reveal a rectifying I–V curve consistent with the formation of a p – n junction. Silicon spheres have been the subject of recent investigations in a broad range of fields spanning mechanics [1] , biotechnology [2] , photonics [3] and green energy [4] . A variety of bottom-up [5] , [6] , [7] and top-down [4] , [8] , [9] methods have been developed to address the need for Si spheres ranging in size from the nm to mm scale. However, to date, no single fabrication methodology exists that is simultaneously scalable in size and quantity over the full spectrum of radii. Recent breakthroughs [10] , [11] , [12] , [13] in harnessing fluidic instabilities [14] , [15] for nanofabrication define a promising direction towards new and scalable methods, but are currently restricted because of the isothermal profile: For example, in cases involving high viscosity-contrast materials systems [14] , [15] , [16] such as Silicon-in-Silica, the isothermal break-up condition [15] would dictate a large break-up wavelength λ T and correspondingly large particles. Here we report on a method for producing Si spheres in a Silica fibre [17] in which capillary break-up is controlled by an axial thermal gradient and a controlled feed speed. In our process, the fibre is fed into a spatially localized flame at a controlled rate, so that melting of the Silicon occurs at a fixed location in space, beyond which a molten Si cylinder cladded by softened Silica develops. Capillary instability causes the core to break-up into a sphere in order to reduce its surface energy. A close analogy is the use of flow rate to control droplet formation in dripping faucets [18] , [19] . By continuously feeding the fibre into the flame a string of particles emerges, the size of which is below that of an isothermal process and approaches the fundamental diameter limit. Challenges in entering the micron-pitch break-up regime The generation of submicron Silicon spheres via a fluid instability mechanism requires very small core diameters to begin with, as the size of the sphere cannot be smaller than (correspondent to wavelength πD —the wavelength equal to the core circumference), where D is the diameter of the core. To generate small cores a multistep process is developed: A 2-mm thick Si rod clad by an 8 mm thick Silica tube is thermally drawn to a Si-core size of 130 μm and redrawn to achieve a core size of 4 μm (see Methods, Supplementary Figs S1 and S2 for details), as shown in Fig. 1a . The resulting twice-drawn fibre is redrawn under high tension in a hydrogen flame. A relatively fast feed speed (3 mm min −1 ) and relatively slow draw speed (15 mm min −1 ) scales the fibre by a factor of while keeping the Si-core intact and without inducing any cracking. This step ( Fig. 1b ) can be repeated multiple times until the desired Si-core diameter is obtained (see Methods, Supplementary Fig. S3 for details). Starting with a 4-μm Si-core fibre, a triple rescaling leads to a continuous Si-core fibre with a diameter of (340±15) nm. 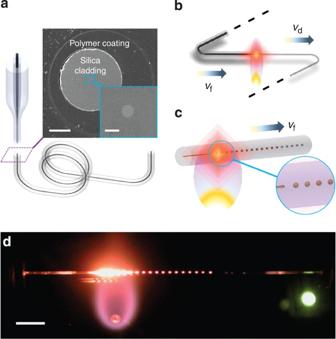Figure 1: Fabrication Process. (a) Schematic representation and experimental results of a redrawn Si-core fibre. (Left scale bar—100 μm, Inset—5 μm). (b) Schematics of a high-tension redraw process that allows, upon repeated application, continuous reduction of the Si-core towards the deep submicron regime. (c) Schematics of our gradual liquefaction technique. (d) Photograph of a typical break-up experiment of 4 μm Si-core fiber under pure hydrogen flow of 0.8 l m−1andvfof 10 μm s−1(scale bar, 5 mm). the break-up period is 1.2 mm and the resulting sphere size is 31 μm. Figure 1: Fabrication Process. ( a ) Schematic representation and experimental results of a redrawn Si-core fibre. (Left scale bar — 100 μm, Inset—5 μm). ( b ) Schematics of a high-tension redraw process that allows, upon repeated application, continuous reduction of the Si-core towards the deep submicron regime. ( c ) Schematics of our gradual liquefaction technique. ( d ) Photograph of a typical break-up experiment of 4 μm Si-core fiber under pure hydrogen flow of 0.8 l m −1 and v f of 10 μm s −1 (scale bar, 5 mm). the break-up period is 1.2 mm and the resulting sphere size is 31 μm. Full size image In the isothermal regime, perturbations to an infinitely long cylinder of diameter D develop into periodic break-up, resulting in a chain of spheres [14] . In the treatment of this problem by Tomotika [15] , an instability growth rate σ(λ) is associated with each perturbation wavelength , the wavelength λ T with the fastest growth rate sets the observed break-up period. λ T depends on the materials’ viscosity ratio, and thus should vary with the chosen temperature. However, for any temperature above the Si melting (1,414 °C) this ratio remains in the 10 8 –10 12 range, resulting in λ T >> πD (see Supplementary Figs S4 and S5 for details). What will happen if the cylinder is neither infinite nor uniformly heated, but instead is dynamically fed into a flame causing the cylinder to melt? We argue that under this condition, droplet formation will occur at the cylinder tip, and that spheres will break off it with a period that is set by the feed speed. If this speed is slow enough, much smaller spheres than those obtained via uniform heating are expected to be formed. Based on this insight, we developed a process in which the fibre is fed through the hot spot of a hydrogen/oxygen flame at a constant speed v f . As predicted, we observed that Si spheres break off of the fibre core one by one at regular intervals, as shown in Fig. 1c,d , respectively (see Supplementary Movie 1 for detailed representation of the process). 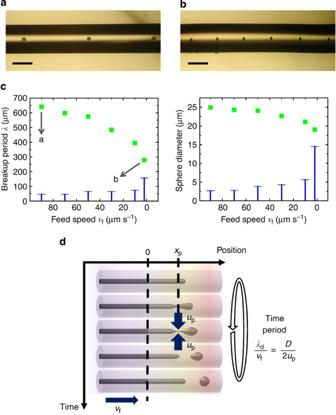Figure 2: Feed speed impact on break-up periods and sphere sizes. (a) Typical high feed speed (vf=90 μm s−1) break-up result in 4 μm Si-core fibre (scale bar, 200 μm). (b) Typical low feed speed (vf=2 μm s−1) break-up result in 4 μm Si-core fibre (scale bar, 200 μm). (c) Break-up periods and corresponding sphere diameters(squares) as a function of the feed speed for the 4 μm Si-core fibre shown together with the magnified graphs of s.d. values (bars) as they appear within each one of the samples. Fibre sections were fed through the hot zone of the hydrogen/oxygen flame at flows of 0.3 and 0.1 l min−1, respectively. In each experiment only the feed speed of the fibre through the flame is varied. The s.d. values in the break-up periods are shown 10-fold magnified while in sphere diameters—1,000-fold magnified. The error in the sphere diameter is assumed to originate from both the break-up period and the fibre core thickness instabilities (seeSupplementary Note 1). (d) Schematic of the step-by-step formation of a sphere and dimensional analysis: in the time it takes to go over one full cycle of sphere formation, in which a lengthλdis fed at speedvf, the core of diameter D is pinched at a speedup. Figure 2a–c show, for a 4-μm Si-core fibre, how slower feed speeds successfully induce the formation of smaller Si spheres. A simple dimensional analysis can account for this scaling of the observed ‘dominant’ break-up period λ d with v f . Indeed, for a given feed speed and in steady state, spheres detach from the Si-core at a fixed location in space: the pinch-off point x = x p . As schematically depicted in Fig. 2d (where x =0 corresponds to the Si melting front), the Si/Silica interfacial tension γ p at x = x p drives the core pinching with a characteristic velocity , where is the local Silica viscosity (see Methods for details). Therefore, λ d is the length of Silicon fed during the time needed for the core to pinch-off, and we can thus write . This expression seemingly implies a linear scaling of λ d with v f , but in reality, x p depends on the feed speed: as v f is increased, pinch-off occurs deeper into the flame, where the higher temperature in turn yields faster pinching speeds. This explains the sub-linear trend of λ d ( v f ) displayed in Fig. 2c . Importantly, with the new technique, the control over v f provides an additional independent knob for tuning the break-up period much more practical than varying the temperature to change the viscosity contrast. This novel control enables, as illustrated in Fig. 2c for this particular example, to reduce the break-up period by a factor of 2 by varying v f , which in turns reduces the spheres diameter by 20%. Figure 2: Feed speed impact on break-up periods and sphere sizes. ( a ) Typical high feed speed ( v f =90 μm s −1 ) break-up result in 4 μm Si-core fibre (scale bar, 200 μm). ( b ) Typical low feed speed ( v f =2 μm s −1 ) break-up result in 4 μm Si-core fibre (scale bar, 200 μm). ( c ) Break-up periods and corresponding sphere diameters(squares) as a function of the feed speed for the 4 μm Si-core fibre shown together with the magnified graphs of s.d. values (bars) as they appear within each one of the samples. Fibre sections were fed through the hot zone of the hydrogen/oxygen flame at flows of 0.3 and 0.1 l min −1 , respectively. In each experiment only the feed speed of the fibre through the flame is varied. The s.d. values in the break-up periods are shown 10-fold magnified while in sphere diameters—1,000-fold magnified. The error in the sphere diameter is assumed to originate from both the break-up period and the fibre core thickness instabilities (see Supplementary Note 1 ). ( d ) Schematic of the step-by-step formation of a sphere and dimensional analysis: in the time it takes to go over one full cycle of sphere formation, in which a length λ d is fed at speed v f , the core of diameter D is pinched at a speed u p . Full size image An alternative viewpoint using the Tomotika model mentioned above can be adopted to qualitatively understand the particle scaling with velocity: In an infinite fluid cylinder perturbations with a wavelength λ grow at a rate σ ( λ ) to break-up on a timescale proportional to 1/ σ ( λ ). In our case, a finite fluid cylinder of length d is fed into the flame at a constant speed v f where d extends from the melting plane of the Silicon, v f and d define an additional timescale d / v f . As a consequence, classical capillary break-up cannot occur for wavelengths with 1/ σ ( λ )<< d / v f , as a wavelength cannot break-up before it is liquefied. For high viscosity contrasts, in which longer wavelengths break-up faster in the Tomotika model (that is, σ is monotonically increasing with λ ), this means that break-up will first occur for the wavelength satisfying 1/ σ ( λ )≈ λ / v f , which will be much smaller than the Tomotika wavelength. Making a quantitative prediction from this model is complicated by the fact that the growth rate σ increases as the fibre is fed deeper into the flame (decreasing the viscosity). One can either use a single ‘typical’ viscosity to estimate σ (which neglects the fact that higher feed speeds will effectively ‘see’ a lower viscosity), or better yet integrate σ ( λ,x ) along an estimated temperature profile T ( x ) ( Supplementary Fig. S6 ) in the fibre until break-up occurs, as described in Supplementary Note 1 , Supplementary Figs S7 and S8 ; either approach can be used to predict particle diameters that are consistent with the observed values to within an order of magnitude. A fundamental difficulty is that the Tomotika growth rate σ ( λ ) is derived for an infinite isothermal cylinder, and is only a crude approximation when applied to our situation, in which the viscosity varies dramatically over the scale of a single λ . Our estimates suggest that the true growth rates are several times larger than the Tomotika model’s, especially for wavelengths on the same scale as the temperature gradient, agreeing with the intuition that temperature non-uniformities can help to accelerate geometric non-uniformities (break-up) compared with Tomotika’s case of a uniform cylinder with only small initial perturbations. In future work, we hope to perform full numerical Stokes simulations with non-uniform viscosities in order to model these effects precisely. Patterning of the core into a necklace of submicron beads Fabrication of 100 nm-scale Si spheres is achieved by first fabricating a fibre with a 23 μm diameter Silica cladding and 325 nm diameter Si-core. This fibre is then fed at 10 μm s −1 through the hot zone of the hydrogen/oxygen flame, while the gas flow rates are set to 0.17 and 0.08 l min −1 , respectively. The typical fibre-embedded Si sphere chain imaged using an optical confocal microscope is shown in Fig. 3a , Supplementary Fig. S9 . The spheres are actually imaged as narrow crosses rather than circular disk patterns. Interestingly, this pattern arises from the astigmatism imposed by the cylindrical lens formed by the fibre surface [20] , [21] . (For aberration-free images refer to Supplementary Fig. S10 .) Note, that the method is not limited to fabrication of submicron spheres but is actually widely scalable as is demonstrated in Supplementary Figs S9, S11 and S12 . The spheres are released from the Silica by etching out the fibre cladding using hydrofluoric acid (HF) and imaged using the scanning electron microscope (SEM) as shown in Fig. 3b,c . Statistical analysis on SEM-imaged spheres reveals that the diameter distribution fits to a normal distribution centered at (460±24) nm, with an average pitch of (1.4±0.3) μm, which is uniform over a cm length scale. Note, that this pitch size is closely approaching the ultimate limit achievable by capillary break-up phenomena— λ = πD =1.1 μm, which is unapproachable by isothermal break-up. Electron backscatter diffraction (EBSD) on a single sphere surface shows a diffraction pattern across the entire sphere meridian suggests the sphere is composed of diamond cubic Silicon, as seen in Fig. 3d . 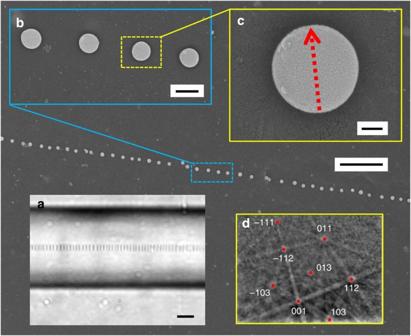Figure 3: Break-up results. The spheres released from the fibre land to the bottom of the container while maintaining the location where they are released. Thus, the resulting chain of spheres mimics the axis of the original fibre (scale bar, 5 μm). Insets depict: (a) Silicon spheres embedded in a Silica fibre as observed using a confocal microscope in transmission mode (scale bar, 5 μm). (b) Enlarged section of the chain giving a sense of the sphere diameter uniformity (scale bar, 0.5 μm). (c) Individual sphere image giving a sense of the sphere shape quality. The dashed red line depicts the meridian along which seven (roughly equally spaced) 20 keV EBSD measurements were performed on a similar sphere. The beginning of the line and arrow tip refer to the location of the first and last measurement, respectively (scale bar, 100 nm). (d) Diffraction pattern averaged from five EBSD measurements (excluding edges) shows good agreement with diamond cubic silicon. Figure 3: Break-up results. The spheres released from the fibre land to the bottom of the container while maintaining the location where they are released. Thus, the resulting chain of spheres mimics the axis of the original fibre (scale bar, 5 μm). Insets depict: ( a ) Silicon spheres embedded in a Silica fibre as observed using a confocal microscope in transmission mode (scale bar, 5 μm). ( b ) Enlarged section of the chain giving a sense of the sphere diameter uniformity (scale bar, 0.5 μm). ( c ) Individual sphere image giving a sense of the sphere shape quality. The dashed red line depicts the meridian along which seven (roughly equally spaced) 20 keV EBSD measurements were performed on a similar sphere. The beginning of the line and arrow tip refer to the location of the first and last measurement, respectively (scale bar, 100 nm). ( d ) Diffraction pattern averaged from five EBSD measurements (excluding edges) shows good agreement with diamond cubic silicon. Full size image To obtain an in-depth understanding of the structure of the Si sphere, a cross-sectional sample was prepared for transmission electron microscopy (TEM) using focused ion beam ( Fig. 4a (inset) ). Selected area electron diffraction of the core of the representative Si sphere reveals that the Silicon is diamond cubic and multi-crystalline ( Fig. 4a ), with several grains comprising the bulk of the volume (see Methods, Supplementary Fig. S13 ) for details). It is well established that the O solubility in equilibrium diamond cubic Si does not exceed fractions of a percent [22] , [23] and that the main origin of O in polycrystalline Si is oxide formation at the grain boundaries [24] , [25] , [26] . To investigate the possible oxide formation at the grain boundaries, we use energy dispersive X-ray spectroscopy (EDX) to qualitatively map the distribution of oxygen within the sphere core ( Fig. 4b , Supplementary Fig. S14 ). EDX line scan does not reveal any increase in the oxygen signal at grain boundaries, indicating that that the oxygen content in the Si-core is below the detection limit of EDX [27] , [28] and that the multi-crystalline Silicon spheres may be sufficiently pristine for electronic applications. An increase in O is observed on the surface of the sphere, consistent with the further TEM observation of an oxide-rich shell forming on the surface, but the deposition of a protective layer of Au-Pd on the surface inhibits further structural characterization of the porous Si on the surface. 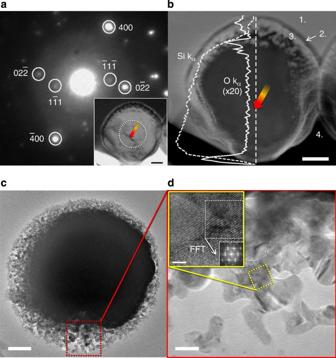Figure 4: Structural and compositional analysis of individual spheres. (a) Selected area electron diffraction pattern, from the region indicated by the dashed circle on the inset, confirming that the core is composed of multiple diamond cubic Silicon grains. Indexed {400}, {022} and {111} spots highlight three distinct grains within the selected region. The inset shows cross-sectional bright-field TEM image of Si sphere prepared using focused ion beam. (b) Dark-field STEM image of the Si sphere cross-section with overlaid EDX line scan. EDX is unable to detect increased oxygen concentration in the Si-core or at the grain boundary (indicated by flame-coloured arrows) visible in the inset ofa(scale bar, 100 nm). Labels indicate deposited protective layers (1: Pt, 2: C, 3: Au and Pd) and four: voids milled by focused ion beam. (c) Bright-field TEM image of a Si sphere, which reveals the core-shell structure (scale bar, 100 nm). (d) Zoomed view of the shell section showing individual Si ‘fingers’ (scale bar, 20 nm). Inset: high-resolution TEM of Si fingers (scale bar, 2 nm). FFT confirms crystallinity and detects multiple grains of diamond cubic Silicon oriented on the [110] zone axis. The measured lattice constant is (0.538±0.008) nm, which is consistent with the literature value 0.543 nm (ref.29). Figure 4: Structural and compositional analysis of individual spheres. ( a ) Selected area electron diffraction pattern, from the region indicated by the dashed circle on the inset, confirming that the core is composed of multiple diamond cubic Silicon grains. Indexed {400}, {022} and {111} spots highlight three distinct grains within the selected region. The inset shows cross-sectional bright-field TEM image of Si sphere prepared using focused ion beam. ( b ) Dark-field STEM image of the Si sphere cross-section with overlaid EDX line scan. EDX is unable to detect increased oxygen concentration in the Si-core or at the grain boundary (indicated by flame-coloured arrows) visible in the inset of a (scale bar, 100 nm). Labels indicate deposited protective layers (1: Pt, 2: C, 3: Au and Pd) and four: voids milled by focused ion beam. ( c ) Bright-field TEM image of a Si sphere, which reveals the core-shell structure (scale bar, 100 nm). ( d ) Zoomed view of the shell section showing individual Si ‘fingers’ (scale bar, 20 nm). Inset: high-resolution TEM of Si fingers (scale bar, 2 nm). FFT confirms crystallinity and detects multiple grains of diamond cubic Silicon oriented on the [110] zone axis. The measured lattice constant is (0.538±0.008) nm, which is consistent with the literature value 0.543 nm (ref. 29 ). Full size image TEM was used to better elucidate the microstructure of the whole Si spheres in addition to SEM imaging in Fig. 3 . A TEM micrograph of a single sphere, shown in Fig. 4c , gives evidence of a porous shell on the sphere surface. The shell is composed of crystalline Si ‘fingers’ ( Fig. 4d ) protruding from the core and is presumably where an interpenetrated Si/Silica mixture formed at the interface between the Si sphere and the Silicon cladding. The material forming the ‘fingers’ was confirmed to be Si by obtaining its lattice constant [29] based on high-resolution TEM images ( Fig. 4d (inset)). We hypothesize that these interpenetrated fingers are either a result of the Si expansion upon crystallizing in a Silica cavity of dimensions that correspond to the liquid Si, in which case the fingers provide a mechanism for stress release, or a result of diffusion of Si into surrounding Silica [30] with consequent precipitation of it into Si nano-clusters [31] due to prolonged thermal treatment or a combination of both. Contact-by-break-up for fabrication of electronic devices In addition to the utility of the gradual-heating approach for nanosphere fabrication, this technique facilitates multicore break-up as a device fabrication tool. In contrast to the uniform-heating method [10] , [11] , which spatially initiate break-up randomly, the local gradual liquefaction inherent to the novel method homogenizes the structural imperfections of the fibre, thus enabling the simultaneous break-up of multiple equal-diameter cores at the same axial position. This allows coherent patterning of multi-cored fibres, in which detachment of droplets from each core occurs in unison. As by conservation of volume the diameter of a sphere is always larger than the cylinder from which it breaks, spheres detaching from multiple closely separated cores can come in contact to form multi-spherical clusters as shown in Fig. 5a schematically for a dual-core Si fibre and confirmed experimentally as shown in Fig. 5b . Specifically, if the distance between multiple cores is smaller than the diameter of the generated spheres, complex structures made of partially merged spheres can be formed (see Methods, Supplementary Fig. S15 for details), a process we coin contact-by-break-up (CBB). 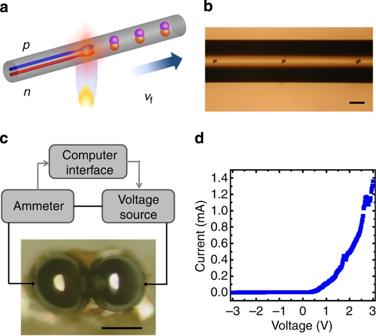Figure 5: Synchronous break-up andp–nmolecule formation. (a) Schematics of break-up of a double-core fibre into bispherical clusters (p- andn-type cores are shown in blue and red, respectively). (b) The resulting chain of bispherical particles as an outcome of process ina(scale bar, 100 μm). (c) Block diagram together with a bispherical pn cluster composed ofn- andp-type spheres, fused together by the simultaneous break-up of two closely separated cores.p-type core has acceptors concentrationNA=6.9 × 1018cm−3and then-type core has donors concentrationND=1.6 × 1019cm−3. High dopants concentrations were chosen so as to ensure satisfactory current conduction through direct contact using tungsten needles (scale bar, 50 μm). (d) I–V curve for the pn diode. Figure 5: Synchronous break-up and p–n molecule formation. ( a ) Schematics of break-up of a double-core fibre into bispherical clusters ( p - and n -type cores are shown in blue and red, respectively). ( b ) The resulting chain of bispherical particles as an outcome of process in a (scale bar, 100 μm). ( c ) Block diagram together with a bispherical pn cluster composed of n - and p -type spheres, fused together by the simultaneous break-up of two closely separated cores. p -type core has acceptors concentration N A =6.9 × 10 18 cm −3 and the n -type core has donors concentration N D =1.6 × 10 19 cm −3 . High dopants concentrations were chosen so as to ensure satisfactory current conduction through direct contact using tungsten needles (scale bar, 50 μm). ( d ) I–V curve for the pn diode. Full size image As a proof-of-concept of the viability of CBB, we fabricate a chain of bispherical pn particles from the break-up of a dual-core fibre comprised of an p -type and an n -type core. Surprisingly, even though the dwell time of the paired pn cluster in the hot zone is much longer than the typical break-up time, we experimentally observe that upon formation, the cluster, as seen in Fig. 5c , does not reshape into a single large sphere. Instead, it remains in the form of a bispherical cluster. This likely results from the presence of the aforementioned mixture layer membrane on the contact surface between the merged spheres, in analogy to the case where two occasionally touching soap bubbles merge into a single ‘double bubble’ with a thin membrane in between [32] . The membrane of interpenetrated Si/Silica composite between the p - and the n -halves of the merged cluster could act as a diffusion barrier for dopants, thus allows maintaining electronic properties of the junction. Without this layer, the dopants would likely completely homogenize over the entire cluster volume. At the same time, this layer remains electrically conductive due to sufficient concentration of crystalline Si. Figure 5d displays the current–voltage characteristics of a pn diode, which clearly displays rectifying behaviour, consistent with the polarity of the device (see Supplementary Note 2 , Supplementary Fig. S16 for details). Post processing of Si-in-Silica multimaterial fibres [33] , [34] using the gradual liquefaction approach enables controlled and scalable production of uniform Si spheres, which can be used on fibres with a wide range of internal core dimensions so as to yield particles from hundreds of nanometres to hundreds of microns. This approach allows to selectively produce spheres that are smaller than their counterpart obtained under uniform heating, despite the large disparity between core and cladding viscosities. These spheres are shown to be comprised of polycrystalline Si with low oxygen content and are surrounded by a porous Si shell. To demonstrate the generality of our approach, a dual-core Si-in-Silica fibre with p - and n -type Si cores is drawn and processed into spheres. The controlled feeding of the fibre in the heat source induces spatially coherent break-up which leads to the joining of the spheres into a bispherical Si ‘ p–n molecule’. The resulting junction is measured to reveal a rectifying I–V curve consistent with the formation of a p–n junction. Preform fabrication and fibre drawing For a preform preparation we use fused quartz tubes and rods by Technical Glass Products and Si rods by Lattice Materials. Typical preform assembly scheme is shown in Supplementary Fig. S1 . First, a Si rod with the diameter of 2 mm is sleeved into a preform with the Silica cladding of 8 mm and drawn at 2,130 °C with v f =1.2 mm min −1 and v d =0.3 m min −1 . This yields a Si-core fibre with the core diameter of 130 μm and the outer diameter of 500 μm. It is then fed into a new preform having Silica cladding diameter of 12 mm and redrawn at 2,095 °C and v f =1.2 mm min −1 , v d =2 m min −1 in order to reduce the Si-core thickness to 4 μm. A typical preform assembly scheme for fibre redraw is shown in Supplementary Fig. S2 . The fibre is protected by an in-line ultraviolet curable coating system. The coating layer is ‘DSM Desotech 3471-3-14(941–314) Desolite single coat coating’ with a thickness of 20–40 μm. At the redraw stage, in order to avoid the break-up of the core material inside the preform before its descent into the fibre, the preform should be fed as fast as possible and drawn as fast as possible, thus shortening the dwell time of Si in the hot zone of the furnace. The fact that only 100–200 μm in the center of the active part of the preform contain material different than silica, allows doing so, while still maintaining a crack-free draw. The feed speed and the draw speed are v f =1.2 mm/ min −1 and v d =2 m min −1 , respectively. The fibre is drawn at lowest possible temperature providing crackless draw (2,095 °C), that is, at the highest possible tension. The redraw of the fibre with a 130-μm Si-core in the conditions described above resulted in 60-m-long continuous section of Si-core fibre, starting from a thin core in the beginning (thinnest sampled was 0.5 μm thick) growing in a few metres and stabilizing at (4±5%) μm. This is roughly the thinnest stably drawable and controllably scalable core size, while using conventional draw process. The redraw of the fibres with ~100 μm Si-core at the conditions described above resulted in continuous-core sections of tens of metres with core sizes of (1.7±50%) μm, and the redraw of the fibres with ~70 μm Si-core has failed to give significantly long sections of fibre with continuous core—these fibres were mostly blank, indicating that the break-up of the core occurred in the preform. Scaling of the fibre core to the nano-metric regime is thus challenging to achieve using conventional fibre-draw techniques [35] , [36] . Conventional techniques are characterized by a ratio of preform feed speed v f to fibre drawing speed v d ranging from two to four orders of magnitude resulting in a typical preform to fibre cross-sectional scaling ratios of few tens to few hundreds. When producing silica fibres, such a v f / v d ratio requires the draw to be performed at relatively low viscosity of silica in order to avoid cracking of the fibre during the draw due to the viscous rupture phenomenon [37] . On the other hand, practical range of scaling ratios limits the core in the preform to diameters that are large enough to prevent the Si break-up to occur in the drawing cone before descending into the fibre, the more so that the high interfacial tension γ =1.5 J m −2 between the core and the cladding [38] speeds up the break-up process. The last would result in a fibre with uneven Si-core of random diameter. Faster feed speed would compensate over this break-up partially, by shortening the dwell time of Si in the drawing cone, where it is sensitive to the capillary instabilities. Unfortunately, this would result in a decreased cross-section scaling ratio, providing a thicker fibre core. To maintain the core thickness unchanged, the draw speed in that case should be increased, which would require an additional decrease in silica viscosity for crack-free fibres. Torch scaling During the first scaling process, the fibre is placed in the hot spot of the flame resulting from the burning of hydrogen flowing at the rate of 0.23 l min −1 through the aperture of the torch outlet having a small diameter of 0.020 inches. Such a small diameter of the outlet aperture is chosen in order to focus the flame and to prevent flashback explosions at this law flow-rate. The 4 μm Si-core fibre was rescaled three times. For each consecutive rescaling iteration the hydrogen flow is reduced by 0.02 l min −1 in order to compensate over the decrease in a heat capacity of the rescaled fibre, so that the high tension conditions can be maintained. Details on the dimensional analysis of gradual-heating break-up As shown in Fig. 2 , when break-up is induced under gradual-heating conditions, the final sphere size can be seen as the result from the competition between the feed speed v f and the velocity u p of the Si/silica interface at the location x p where the core periodically pinches-off. We give here more details on how the expression of u p given in the main body of the paper is obtained. We can approach the question of the velocity of the interface through dimensional analysis and scaling of the governing fluid mechanics equations. Fluid flow in the system is predominantly forced by interfacial tension; therefore, the relevant boundary condition to focus on is the normal stress balance at the Si/silica interface, which writes: where and T Si are the stress tensors in silica and Si, respectively, and γ is the Si/silica interfacial tension. The components of the stress tensor in Si are: where v i are the components of the velocity field in Si, and p Si is the pressure field in Si. A similar expression holds for silica. Assuming low-Reynolds number flows in both Si and silica, and noting that the characteristic length scale in the problem is the Si-core diameter D , we conclude that the characteristic pressures at the pinch-off location are and , respectively, in Si and silica. At that point, the stress balance condition can be rewritten: As shown in Supplementary Fig. S4 , under all practical temperatures, , which allows us to simplify the previous equation and obtain the expression for u p used in the main text: From this approach, we can compute Reynolds numbers for Si and silica: and . For any practical pair ( D , T ) considered, these Reynolds numbers are both always orders of magnitude below unity, which validates the approximation of Stokes flow regime leading to the scaling of characteristic pressure in the fluids made above. TEM sample preparation and TEM measurements details Investigation of the sphere structure included the inspection of the bare spheres directly released on the Cu-frame carbon membrane TEM grid. To prepare the sample the fibre section is immobilized on CF300-CU CARBON FILM on 300 Cu mesh copper grid by Electron Microscopy Sciences (3 mm in diameter), then immersed in HF. It allowed an observation of core-shell structure comprising the sphere shown in Fig. 4c . Further investigation included focused ion beam sectioning [39] of the spheres using FEI Helios NanoLab 600, and high-resolution transmission electron microscope (HR-TEM) structural analysis on JEOL 2010FEG TEM operated at 200 kV, including large area electron diffraction ( Supplementary Fig. S13 ), and EDX ( Supplementary Fig. S14 ). Structural analysis and the electron diffraction patterns reveal that the core is comprised of a small numbers [3] , [4] , [5] of monocrystalline grains mediated by thin trenchant boundaries. The EDX analysis reveals that the level of oxygen in the core is comparable to typical electronic-grade Si reading (for comparison see Nishimura [40] ). Bispherical p–n junction fabrication First, a preform containing two separated Si rods was prepared and drawn into a double-core fibre. One p -type Si rod (electron acceptors concentration N A =6.9 × 10 18 cm −3 ) and one n -type Si rod (electron donors concentration N D =1.6 × 10 19 cm −3 ) with the diameter of 2 mm were sleeved into a preform with a silica cladding of 12 mm, and drawn at 2,130 °C with the feed speed v f =0.6 mm min −1 and draw speed v d =0.6 m min −1 . Then a section of the resulting fibre was incorporated into a new preform in a similar fashion as described in Supplementary Fig. S1 . The preform was then drawn with the feed speed v f =1.2 mm min −1 and the draw speed v d =1.2 m min −1 at the draw temperature of 2,085 °C. The resulting fibre cross-section is shown in Supplementary Fig. S15 . The cross-sectional geometry is maintained exactly as in the preform. The core separation is preserved, and both cores have the same diameter of 23 μm. A section of a dual-core fibre underwent the gradual-heating break-up at a feed speed v f =20 μm s −1 using a flame resulting from gas flows of hydrogen and oxygen of 0.42 l min −1 and 0.20 l min −1 , respectively, resulting in a chain of in-fibre bispherical p–n junctions in a similar manner as shown in Fig. 5b . The bispherical p–n junctions were released from the fibre by dissolving silica cladding in HF acid as appear in Fig. 5c . Current-voltage characteristics measurement of the p–n junction After a two-sphere particle is released out of the fibre cladding using HF acid, two tungsten needles (2.4 μm, Cascade Microtech, PTT-24-25) are brought in contact with the spheres’ surface using manual probe positioners (Cascade Microtech). Voltage is applied between the probes by a Keithley 6517A Electrometer while current is measured by a Keithley 6487 Picoammeter, both units controlled via a LabView custom interface. For further details see Supplementary Note 2 , Supplementary Fig. S16 . How to cite this article: Gumennik, A. et al. Silicon-in-silica spheres via axial thermal gradient in-fibre capillary instabilities. Nat. Commun. 4:2216 doi: 10.1038/ncomms3216 (2013).